The Glanville fritillary genome retains an ancient karyotype and reveals selective chromosomal fusions in Lepidoptera Previous studies have reported that chromosome synteny in Lepidoptera has been well conserved, yet the number of haploid chromosomes varies widely from 5 to 223. Here we report the genome (393 Mb) of the Glanville fritillary butterfly ( Melitaea cinxia ; Nymphalidae), a widely recognized model species in metapopulation biology and eco-evolutionary research, which has the putative ancestral karyotype of n =31. Using a phylogenetic analyses of Nymphalidae and of other Lepidoptera, combined with orthologue-level comparisons of chromosomes, we conclude that the ancestral lepidopteran karyotype has been n =31 for at least 140 My. We show that fusion chromosomes have retained the ancestral chromosome segments and very few rearrangements have occurred across the fusion sites. The same, shortest ancestral chromosomes have independently participated in fusion events in species with smaller karyotypes. The short chromosomes have higher rearrangement rate than long ones. These characteristics highlight distinctive features of the evolutionary dynamics of butterflies and moths. Butterflies and moths (Lepidoptera) have a large number of short holocentric chromosomes [1] , [2] , [3] with substantial variation in chromosome number [4] , [5] , [6] ( n =5–223). However, the most common chromosome numbers are n =29–31 (refs 7 , 8 ), and the distribution is markedly skewed with only a few species having n >31. The ancestral chromosome number has been inferred to be 31 (refs 9 , 10 ), but until recently this has been difficult to confirm due to lack of comprehensive phylogenies. In spite of much variation in the number of chromosomes, the amount of DNA is approximately the same in different species, suggesting that species with fewer chromosomes have, on average, longer chromosomes [7] . Lepidopteran karyotypes are thought to have evolved via fusion and fission events [7] . Due to the holocentric chromosome structure with dispersed kinetochore activity, such events have been expected to be less deleterious than in monocentric chromosomes [11] , [12] . Conversely, holocentricity may restrict gene flow [13] through meiotic [14] and recombination suppression mechanisms [15] . Detailed sequence-level studies of structural variation in lepidopteran chromosomes became feasible with the publication of the whole-genome sequence of Bombyx mori ( n =28) [16] . Paradoxically, in spite of their holocentric chromosome structure, genomic comparison of Heliconius melpomene ( n =21) with B. mori suggested a highly conserved chromosomal gene content and an ancestral chromosome number of n =31 (ref. 10 ), supporting previous low-resolution comparisons in other lepidopteran species [17] , [18] , [19] , [20] , [21] , [22] , [23] , [24] . Linkage maps suggest that the karyotypes of B. mori and H. melpomene have evolved via several fusion events. Potential fusion chromosomes have been identified in both species [10] , [21] , [22] , [25] , but confirmation has not been possible without a whole-genome sequence and a high-density linkage map for a species with the putative ancestral karyotype. Here we describe the genome of the Glanville fritillary butterfly ( Melitaea cinxia ), the first butterfly species with n =31 and for which both the genome and a high-density linkage map [26] are now available. Our analysis of chromosome fusions in B. mori and H. melpomene suggests unexpected features shaping karyotype evolution in Lepidoptera. Sequencing of the M. cinxia genome was based on samples from a polymorphic natural population ( Supplementary Note 1 ), as the yield of DNA from a single individual was insufficient and no inbred lines were available ( Supplementary Note 2 ). The initial 393 Mb assembly of the genome was performed using 454 and Illumina paired-end (PE) reads from a single male and Illumina PE reads from a pool of 10 full-sibs ( Supplementary Notes 2 and 3 ). 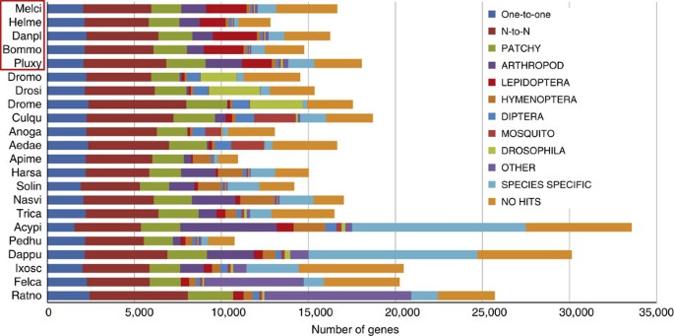Figure 1: Number of proteins in different classes of orthologous groups. The statistics forM. cinxiaare very similar to those for other Lepidoptera, including 5,977 conserved core proteins, 7,177 taxonomic order-, family- or species-specific proteins and 3,513 proteins without detectable sequence similarity to others. There appears to be rapid turnover of gene content in the genomes, indicated by the large proportion of order- and family-specific groups, which represent either rapidly evolving genes or dispensable ancient paralogues that have been deleted from most other lineages. Species codes are as used in SwissProt: Melci=Melitaea cinxia, Helme=Heliconius melpomene, Danpl=Danaus plexippus, Bommo=Bombyx mori, Pluxy=Plutella xylostella, Dromo=Drosophila mojavensis, Drosi=Drosophila simulans, Drome=Drosophila melanogaster, Culqu=Culex quinquefasciatus, Anoga=Anopheles gambiae, Aedae=Aedes aegypti, Apime=Apis mellifera, Harsa=Harpegnathos saltator, Solin=Solenopsis invicta, Nasvi=Nasonia vitripennis, Trica=Tribolium castaneum, Acypi=Acyrthosiphon pisum, Pedhu=Pediculus humanus, Dappu=Daphnia pulex, Ixosc=Ixodes scapularis, Felca=Felis catusand Ratno=Rattus norvegicus.The lepidopteran species are highlighted with a box. SeeSupplementary Note 8for the definition of classes. The contigs were then scaffolded [27] with PE and mate-pair (MP) library data from several full-sib families and an unrelated individual, which were sequenced with SOLiD, Illumina and 454 platforms ( Supplementary Figs 1–3 ; Supplementary Table 1 ). The final assembly of the nuclear genome comprises 49,851 contigs (N50=13 kb) and 8,262 scaffolds (N50=119 kb), with an overall coverage of 95 × ( Supplementary Figs 4–6 ; Supplementary Tables 1 and 3 ). A linkage map based on 40,718 single nucleotide polymorphisms (SNPs) [26] assigned 3,507 scaffolds (318 Mb) to 31 linkage groups, matching the 31 chromosomes reported for this species in a cytogenetic study [28] ( Supplementary Table 6 ; Supplementary Note 5 ). For subsequent superscaffolding, we applied an in-house method utilizing the linkage map, long MP data and PacBio reads. The resulting 1,453 superscaffolds (N50=331 kb) cover 72% of the genome ( Supplementary Fig. 7 ; Supplementary Tables 4 and 5 ). 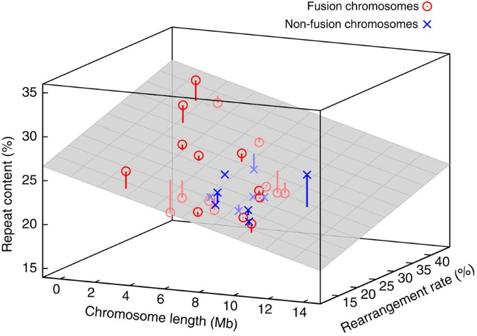Figure 6: Relationships among chromosome length, chromosome rearrangement rate and percentage of repetitive elements in the 31 chromosomes ofMelitaea cinxia. The rearrangement rate is described by the number of chromosomal breakpoints scaled by the number of orthologues. A plane minimizing squared error was fitted to the data and is shown in grey. Drop lines are drawn from each point to this plane. The remaining 4,846 scaffolds covering 111 Mb lack consistent map information. The mitochondrial genome (15,171 bp) was assembled and annotated separately ( Supplementary Figs 8 and 13 ; Supplementary Tables 23 and 24 ; Supplementary Notes 3 and 8 ). The quality of the assembly was assessed using several approaches and data sets, including PE, MP and PacBio read data and independently assembled transcriptome data, which were mapped to genomic contigs and scaffolds ( Supplementary Note 6 ). Estimates of genome completeness and correctness indicate that the assembly is of high quality ( Supplementary Figs 9 and 10 ; Supplementary Tables 7–14 ). Most importantly, the scaffolds show high consistency with the linkage map (91.4% non-chimeric scaffolds). The quality of the superscaffolds was assessed by comparison with an independent high-density linkage map, which showed that only 2.4% of superscaffolds have short chimeric stretches, mostly at their ends. We predicted 16,667 gene models, the vast majority of which (96%) were supported by transcriptome data ( Supplementary Tables 2, 17 and 18 ; Supplementary Note 8 ). Clustering the protein sequences into orthologous groups shows that, consistent with previous reports [29] , the sequenced lepidopteran genomes have very similar gene content despite 140 My [30] of independent evolution ( Fig. 1 , Supplementary Figs 17–19 ). Functional annotations were performed separately for the predicted gene models and the assembled transcripts, yielding protein descriptions and gene ontology (GO) classifications for 12,410, KEGG pathways for 3,685 and InterProScan hits for 8,529 gene models ( Supplementary Figs 14–16 ). We identified noncoding RNA genes including miRNA precursors, ribosomal RNAs, transfer RNAs and spliceosomal small nuclear RNAs ( Supplementary Figs 11 and 12 , Supplementary Tables 19–22 ). 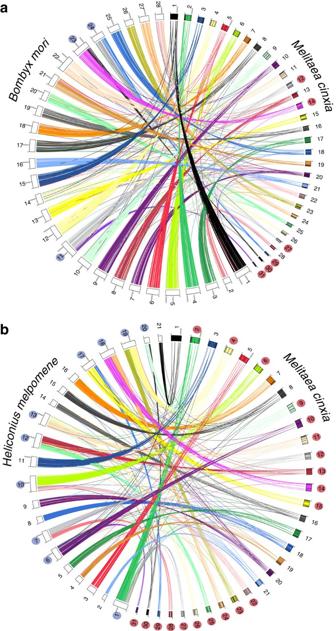Moreover, we carried out manual curation of gene models and descriptions for 558 genes ( Supplementary Fig. Figure 2: Chromosome mapping ofMelitaea cinxiatoBombyx moriandHeliconius melpomene. (a) One-to-one orthologues (4,485) connectingM. cinxiaandB. morichromosomes and (b) 3,869 one-to-one orthologues connectingM. cinxiaandH. melpomenechromosomes.M. cinxiachromosomes are numbered according to chromosome length from the largest to the smallest. The links leading fromM. cinxiachromosomes are pooled into bins that are ordered within chromosomes. Bands drawn inM. cinxiachromosomes represent bin borders. Chromosome 1 is the Z chromosome inM. cinxiaandB. mori. The fusion chromosomes are shaded with blue and the orthologous chromosomes inM. cinxiawith red. 20 ; Supplementary Table 25 ; Supplementary Data 1 ), including the Hox gene cluster. We identified all canonical Hox genes and four copies of the special homeobox ( Shx ) genes, two ShxA , and one ShxB and C ( Supplementary Figs 21 and 22 ; Supplementary Note 8 ). All the Hox genes follow the gene order and location described for other Lepidoptera, but the duplication of ShxA and lack of ShxD are distinct from other nymphalid butterflies [10] , [31] . Figure 1: Number of proteins in different classes of orthologous groups. The statistics for M. cinxia are very similar to those for other Lepidoptera, including 5,977 conserved core proteins, 7,177 taxonomic order-, family- or species-specific proteins and 3,513 proteins without detectable sequence similarity to others. There appears to be rapid turnover of gene content in the genomes, indicated by the large proportion of order- and family-specific groups, which represent either rapidly evolving genes or dispensable ancient paralogues that have been deleted from most other lineages. Species codes are as used in SwissProt: Melci= Melitaea cinxia , Helme= Heliconius melpomene , Danpl= Danaus plexippus , Bommo= Bombyx mori , Pluxy= Plutella xylostella , Dromo= Drosophila mojavensis , Drosi= Drosophila simulans , Drome= Drosophila melanogaster , Culqu= Culex quinquefasciatus , Anoga= Anopheles gambiae , Aedae= Aedes aegypti , Apime= Apis mellifera , Harsa= Harpegnathos saltator , Solin= Solenopsis invicta , Nasvi= Nasonia vitripennis , Trica= Tribolium castaneum , Acypi= Acyrthosiphon pisum , Pedhu= Pediculus humanus , Dappu= Daphnia pulex , Ixosc= Ixodes scapularis , Felca= Felis catus and Ratno= Rattus norvegicus. The lepidopteran species are highlighted with a box. See Supplementary Note 8 for the definition of classes. Full size image Genomic variation was characterized with three independent data sets ( Supplementary Figs 23 and 24 ; Supplementary Tables 26 and 27 ; Supplementary Note 9 ). In a group of 10 full-sibs and an independent individual sequenced with Illumina, more than five million SNPs were identified corresponding to an average density of 13.2 SNPs per kb. The SNP density was 8.2 SNPs/kb in the coding exons, which is roughly half of the density in introns (15.3 SNPs per kb). Approximately half a million indels with an average density of 1.7 per kb were identified. Longer indel variants (>50 bp) were detected using the PacBio data comprising 2,165 deletions and 313 insertions. We have described elsewhere genetic variation in four regional metapopulations of M. cinxia using extensive RNA-seq data [32] . While the GC content varies among Lepidoptera ( Supplementary Table 18 ), the average GC content of the M. cinxia genome (33%) is distributed remarkably uniformly across all the chromosomes, similarly to that found in B. mori ( Supplementary Figs 26, 27, 30 and 31 ; Supplementary Note 10 ). The median gene density is 3 per 100 kb in both species ( Supplementary Fig. 28 ). Uniform GC and gene content distributions across the chromosomes are characteristics of species with holocentric chromosomes [33] , [34] , [35] , [36] , contrasting with species that have monocentric chromosomes with localized centromeres, in which the genome is compartmentalized to GC-rich and GC-poor regions with higher and lower gene densities [37] . Repetitive elements comprise 28% of the assembled M. cinxia genome ( Supplementary Tables 15 and 16 ; Supplementary Note 7 ). The proportion of repetitive elements fluctuates across the chromosomes from 7 to 42% within 100 kb sliding windows ( Supplementary Figs 29–31 ), but it does not show a clear pattern. The distribution of repeats is strikingly different from that in human and mouse, which have a high repeat content in the pericentromeric and subtelomeric regions [38] , but it also differs from holocentric nematodes, in which repeats are enriched in distal chromosome regions [34] , [35] . With this study, a whole-genome sequence and a high-resolution linkage map are available for three lepidopteran species, M. cinxia , B. mori [16] , [17] and H. melpomene [10] , [39] . In interspecific chromosomal comparisons, 4,485 one-to-one orthologous genes with map information were identified between M. cinxia and B. mori , and 3,869 between M. cinxia and H. melpomene . The majority (96%) of these orthologues mapped to orthologous chromosomes among the three species ( Fig. 2 ; Supplementary Tables 28 and 29 ; Supplementary Note 11 ). The remaining 4%, representing putative translocated genes, were relatively evenly distributed and comprise <6% of the genes on any chromosome ( Supplementary Figs 33–35 ; Supplementary Note 12 ). Comparison of M. cinxia with other lepidopteran species carrying the putative ancestral chromosome number of n =31, namely, Plutella xylostella [40] and Biston betularius [22] ( Figs 3a and 4 ), together with the results of previous studies [21] , [22] , [23] , confirms that overall chromosome synteny has been strikingly well conserved in all 31 chromosomes among distantly related (>140 My) [30] Lepidoptera ( Supplementary Tables 30–32 ; Supplementary Note 11 ). The phylogenetic range covers almost all Ditrysia and thus represents at least 95% of existing species ( Fig. 3a ). The distribution of karyotypes on a phylogeny of 312 species in the family Nymphalidae ( Fig. 3b ; Supplementary Fig. 32 ; Supplementary Note 11 ; Supplementary Data 2 ) further indicates that n =31 is unambiguously the ancestral karyotype in this family, although there are some subfamilies (for example, Danainae and Satyrinae) that show much variation in chromosome number even among closely related lineages. Our data argue against the suggestion [7] that repeated fusion and fission events followed by selection would have maintained the n =31 karyotype in Lepidoptera (see also Saura et al. [6] ). Rather, the results indicate that high macrosynteny is a manifestation of the exceptional stability of the ancestral karyotype [18] , [22] , [23] . Figure 2: Chromosome mapping of Melitaea cinxia to Bombyx mori and Heliconius melpomene. ( a ) One-to-one orthologues (4,485) connecting M. cinxia and B. mori chromosomes and ( b ) 3,869 one-to-one orthologues connecting M. cinxia and H. melpomene chromosomes. M. cinxia chromosomes are numbered according to chromosome length from the largest to the smallest. The links leading from M. cinxia chromosomes are pooled into bins that are ordered within chromosomes. Bands drawn in M. cinxia chromosomes represent bin borders. Chromosome 1 is the Z chromosome in M. cinxia and B. mori . 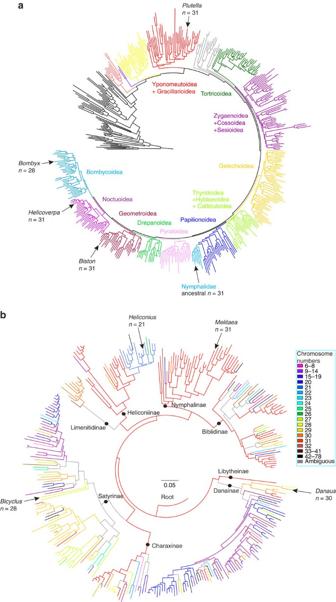The fusion chromosomes are shaded with blue and the orthologous chromosomes in M. cinxia with red. Figure 3: Haploid chromosome numbers mapped onto the lepidopteran tree of life and a phylogenetic hypothesis for Nymphalidae. (a) The lepidopteran tree of life showing the placement of focal species with their haploid chromosome number (n). The named species are those for which whole-genome sequence and linkage map are available (only linkage map forBiston). Major clades, often defined as superfamilies, are coloured. In the Papilionoidea clade (the butterflies), the family Nymphalidae is highlighted in light blue, with the putative ancestral chromosome number ofn=31 (for justification see panelb). The topology is taken from Regieret al.69(b) Haploid chromosome number mapped onto a phylogenetic hypothesis for Nymphalidae. The character state ‘31’ is shown to be the most likely ancestral state for the family. The four species with whole-genome sequences are highlighted. Details of the source of phylogenetic hypothesis as well as chromosome numbers are found in theSupplementary Note 11. Full size image Figure 3: Haploid chromosome numbers mapped onto the lepidopteran tree of life and a phylogenetic hypothesis for Nymphalidae. ( a ) The lepidopteran tree of life showing the placement of focal species with their haploid chromosome number ( n ). The named species are those for which whole-genome sequence and linkage map are available (only linkage map for Biston ). Major clades, often defined as superfamilies, are coloured. In the Papilionoidea clade (the butterflies), the family Nymphalidae is highlighted in light blue, with the putative ancestral chromosome number of n =31 (for justification see panel b ). The topology is taken from Regier et al. [69] ( b ) Haploid chromosome number mapped onto a phylogenetic hypothesis for Nymphalidae. The character state ‘31’ is shown to be the most likely ancestral state for the family. The four species with whole-genome sequences are highlighted. 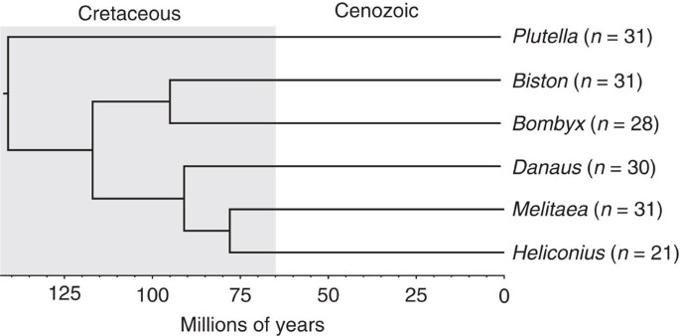Details of the source of phylogenetic hypothesis as well as chromosome numbers are found in the Supplementary Note 11 . Figure 4: The chronogram of the lepidopteran species for which the whole-genome sequence or linkage map, or both, are available together with haploid chromosome numbers. Times of divergence forDanaus,HeliconiusandMelitaeaare taken from Wahlberget al.70, the other times of divergence are from Wahlberget al.30. Full size image Figure 4: The chronogram of the lepidopteran species for which the whole-genome sequence or linkage map, or both, are available together with haploid chromosome numbers. Times of divergence for Danaus , Heliconius and Melitaea are taken from Wahlberg et al. [70] , the other times of divergence are from Wahlberg et al. [30] . Full size image The M. cinxia genome allows us to identify potential fusion and fission events that have shaped the B. mori ( n =28) and H. melpomene ( n =21) genomes from the ancestral karyotype. Our data confirm 3 fusion events in B. mori and 10 fusions in H. melpomene [10] , [22] ( Figs 2 and 5 ; Supplementary Figs 36 and 37 ; Supplementary Note 12 ). A prominent feature of the fusions in both species is the participation of the shortest orthologous M. cinxia chromosomes (chrs 29–31 and 22–31 in B. mori and H. melpomene fusions, respectively; Fig. 2 ). The bias towards the shortest chromosomes is highly significant, P =0.001. Reconstruction of the fusion chromosomes revealed that four of the H. melpomene fusions are lineage specific ( Fig. 2 ; Fig. 5a ). Surprisingly, the six ancestral chromosomes participating in the fusion events in B. mori are also involved in H. melpomene fusions, albeit with non-orthologous fusion partners ( Fig. 5b ), suggesting a preference for a subset of chromosomes to participate in fusion events in evolutionarily distant lineages. The probability of the same six chromosomes being involved in independent fusion events in the two species by chance is low, P =0.05. 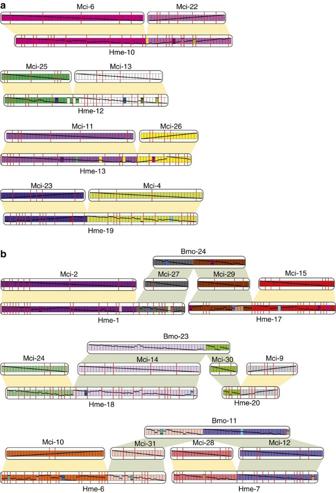These results suggest that selection favours a subset of possible fusion events, possibly at the level of chromosome segregation or through the hypothetical sequence elements associated with the shortest chromosomes. Figure 5:Melitaea cinxiachromosomes involved in fusion events inBombyx moriandHeliconius melpomene. (a) Fusions unique toH. melpomene.(b) Fusions in which the sameM. cinxiaorthologous chromosomes have been fused in bothB. moriandH. melpomene. Each box represents one superscaffold inM. cinxiaand a scaffold inH. melpomene.The colour of each box is derived from the chromosomal origin of the orthologous segment in theM. cinxiagenome (compare withSupplementary Fig. 36). Horizontal lines within the boxes show the corresponding loci inM. cinxiachromosomes, and red vertical lines show recombination sites (bin boundaries) in the linkage map. Figure 5: Melitaea cinxia chromosomes involved in fusion events in Bombyx mori and Heliconius melpomene . ( a ) Fusions unique to H. melpomene. ( b ) Fusions in which the same M. cinxia orthologous chromosomes have been fused in both B. mori and H. melpomene . Each box represents one superscaffold in M. cinxia and a scaffold in H. melpomene. The colour of each box is derived from the chromosomal origin of the orthologous segment in the M. cinxia genome (compare with Supplementary Fig. 36 ). Horizontal lines within the boxes show the corresponding loci in M. cinxia chromosomes, and red vertical lines show recombination sites (bin boundaries) in the linkage map. Full size image A preference for short chromosomes in fusions may be related to a negative relationship between the rate of intrachromosomal rearrangement and chromosome length in M. cinxia ( Fig. 6 ; r =−0.48, P =0.007), in which chromosome length is furthermore inversely related to the percentage of repetitive sequence ( r =−0.73, P <2.8e−6). These relationships imply that longer chromosomes containing fewer repetitive elements are more stable and have fewer intrachromosomal rearrangements, whereas shorter chromosomes are more prone to elevated inter- and intrachromosomal rearrangement. This result is in agreement with the observation that 7 out of the 11 chromosomes with the strongest indication of introgression between four species of Heliconius butterflies [10] are fusion chromosomes. Figure 6: Relationships among chromosome length, chromosome rearrangement rate and percentage of repetitive elements in the 31 chromosomes of Melitaea cinxia . The rearrangement rate is described by the number of chromosomal breakpoints scaled by the number of orthologues. A plane minimizing squared error was fitted to the data and is shown in grey. Drop lines are drawn from each point to this plane. Full size image The putative fusion regions in B. mori show 4% higher abundance of retrotransposons compared with the whole genome ( Supplementary Tables 33 and 34 ; Supplementary Note 12 ). This may reflect the persistence of retrotransposons at ancient telomere sites, given the role of the LINE and PLE elements in telomere maintenance [41] , [42] , but also a possible role for retrotransposons in facilitating the fusion process [43] . It is noteworthy that even though the same six orthologous chromosomes have participated in the fusions in B. mori and H. melpomene , the orientation of the chromosomes is different between the two species in two of the three cases ( Fig. 5b ; Supplementary Fig. 36 ). Comparing the B. mori and H. melpomene fusion chromosomes with the orthologous M. cinxia non-fused chromosomes, we observe that once the fusion event took place, there was very little further rearrangement across the fusion site, with a sharp boundary separating the fused chromosomes ( Fig. 5 ; Supplementary Figs 36 and 37 ). Thus, no orthologous genes have crossed the fusion boundary in B. mori , and only 13 such events were detected in H. melpomene over 10 chromosomes. The reference genome of the Glanville fritillary, featuring the ancient karyotype with n =31, provides new insight into karyotype evolution in Lepidoptera. Comparisons between M. cinxia , B. mori and H. melpomene suggest that lepidopteran chromosomal fusion events favour the shortest chromosomes, which have high rates of chromosomal evolution and high frequency of transposable elements (TEs). The fusion chromosomes retain the ancestral chromosome segments and gene content with very little rearrangement across sharp fusion boundaries. Features such as conserved gene content in chromosomes and constrained fusions offer practical advantages for further lepidopteran genomic studies, by providing a guide for scaffolding and validation of newly sequenced genomes. These characteristics emphasize the distinctive features of evolutionary dynamics in holocentric chromosomes of butterflies and moths, which appear to evolve in a different manner than most other metazoan genomes. Samples and sequencing Initial sequencing of genomic DNA ( Supplementary Note 2 ) was carried out using a single male larva collected from the Åland Islands, Finland. A male larva was used to avoid sequencing of the female W chromosome known to have high repetitive sequence content [44] , [45] . In addition, a single female larva was used for sequencing of mitochondrial DNA (mtDNA). DNA was extracted using modified glass rod spooling methods. The male sample was used for the production of several 454 single-read fragment libraries, and 454 sequencing was carried out according to the manufacturer’s instructions, and subsequently used for contig assembly. In the sequencing of PE and MP libraries ( Supplementary Note 2 ), we used a single male sample and several sets of 10–100 full-sibs to obtain a sufficient yield of high-molecular-weight DNA for library preparation ( Supplementary Table 1 ). PE and MP data were produced using Illumina, SOLiD (ABI) and 454 (Roche) platforms and used for scaffolding ( Supplementary Fig. 1 ). PE data consisted of Illumina libraries with insert size of 500 and 800 bp. The MP data included Illumina and SOLiD libraries with insert sizes of 1, 2, 3 and 5 kb, and 454 libraries with insert sizes of 8 and 16 kb ( Supplementary Fig. 3 ; Supplementary Table 1 ). DNA for the short-insert (≤1 kb) libraries was extracted from thorax tissues using NucleoSpin Tissue Kits. For the long-insert (>1 kb) MP libraries and PacBio sequencing, DNA was extracted from pools of thorax or abdomen tissues using the CsCl purification method [46] , which was modified to increase the yield, integrity and purity of DNA ( Supplementary Fig. 2 ). The Illumina PE libraries were prepared according to Tuupanen et al. [47] but using PE adapters and larger size selection, and sequenced with an Illumina Genome Analyzer IIx (500 bp library) or a HiSeq 2000 (800 bp library) following standard PE-sequencing protocols. SOLiD and Illumina MP libraries were produced as described by the manufacturer (SOLiD MP library kit, Life technologies, CA, USA) with in-house modifications, and sequenced using SOLiD 5500XL and HiScan SQ. The 454 MP libraries were constructed by Roche 454 Life Sciences Sequencing Services (Branford, CT, USA) and sequenced with 454 FLX. Libraries for PacBio sequencing were constructed following the manufacturer’s protocols, and run on PacBioRS. Transcriptome data from RNA-seq experiments were used in gene prediction, functional annotation and variation and linkage disequilibrium (LD) analyses ( Supplementary Table 2 ; Supplementary Note 2 ). For gene prediction and functional annotation, we used pooled abdomen and mixed tissue samples consisting of head, thorax and larval tissues. For variation analyses, only thorax samples were used. RNA was extracted using the Trizol method (Life Technologies) followed by acid phenol–chloroform–isoamyl alcohol and chloroform extractions. RNA-sequencing libraries for the pooled samples were constructed using the Illumina TruSeq RNA Sample Preparation kit (A) and sequenced with Illumina HiSeq 2000 according to the manufacturer’s instructions. For the variation analyses, two RNA-seq libraries were prepared for each individual using an in-house polyA-anchoring-based RNA-seq library protocol ( Supplementary Note 2 ). These libraries were sequenced according to the manufacturer’s instructions with Illumina HiSeq 2000 and HighScan SQ sequencers using the PE mode. Genome assembly Before the assembly, raw reads were filtered and trimmed as described in Supplementary Note 3 . To correct sequencing errors and to eliminate additional variation from heterogenous DNA samples, we used two in-house error-correction methods, Coral [48] for 454 and Illumina reads, and HybridSHREC [49] for SOLiD colour-space reads. Error-corrected 454 and Illumina PE reads were assembled using Newbler (Roche) and SOAPdenovo [50] ( Supplementary Note 3 ). Contigs with a minimal length of 500 bp were used in scaffolding. For scaffolding, we used in-house MIP Scaffolder software [27] , and required at least two read pairs for connecting a pair of contigs. Scaffolding was performed in seven stages in which the PE and MP libraries were added in ascending order of insert size. The most substantial increase in the N50 was observed with the 16 kb 454 MP library ( Supplementary Fig. 4 ). After scaffolding, we used Illumina PE libraries to close the gaps between the contigs using SOAPdenovo GapCloser [50] . Only scaffolds longer than 1,500 bp were included into the final scaffold set. Ribosomal DNA and mtDNA were assembled separately using contigs, which were excluded from genome scaffolding due to their high abundance ( Supplementary Note 3 ). In addition, assembly of 454 reads from a single female was used in the assembly of mtDNA. To increase the continuity of the genome assembly, we constructed superscaffolds using an in-house-developed method that utilizes the linkage map, MP and PacBio data ( Supplementary Note 3 ). First, MP reads and PacBio reads were aligned against existing scaffolds using BWA [51] and an in-house SANS aligner [52] , respectively. After subsequent filtering, the linkage map was used as a guide to determine the most reliable path between the scaffolds to yield individual superscaffolds. Linkage map The linkage map for M. cinxia has been described by Rastas et al. [26] and in Supplementary Note 5 . For the purpose of validating the superscaffolds, another linkage map was constructed by a similar procedure as in Rastas et al. [26] using 12,109 SNPs from an independent full-sib family with 19 offspring. Genome validation Correctness and consistency of the genomic assembly were assessed using eight approaches ( Supplementary Table 7 ; Supplementary Note 6 ). (1) Correctness of the contigs was assessed by mapping PE and MP reads to the genome, and calculating the concordant mappings. (2) Correctness of the scaffolds was evaluated by re-scaffolding the contigs using PacBio reads and calculating the contig joins concordant with the scaffolds. (3) Consistency of the scaffolds was estimated by counting non-chimeric scaffolds based on the linkage map. (4) Completeness of the genome was evaluated by aligning assembled transcripts to scaffolds and calculating the proportion of aligned transcripts. (5) Completeness was further assessed by estimating the proportion of conserved core genes found in the genome and (6) the level of sequence synteny among other lepidopteran species. (7) Correctness and consistency of the superscaffolds were assessed by comparing gene order against B. mori within superscaffolds and (8) by estimating the proportion of non-chimeric scaffolds using an independent linkage map. Prediction of repetitive elements M. cinxia -specific TEs were predicted de novo as described in Supplementary Note 7 . Long terminal repeat retrotransposons were searched using LTR_Finder [53] . The predicted TEs of M. cinxia were combined with the RebBase (v. 20120418) library of consensus TEs from different species [54] . The consensus sequences of TE families were collected as a M. cinxia repeat library and annotated using Repbase18.05, RepeatPeps [54] and Dfam 1.1 (ref. 55 ) databases. RepeatMasker-open-4-0-2 (Smit, A.F.A., Hubley, R. and Green, P. RepeatMasker at http://repeatmasker.org ) was used to estimate the distribution of TEs and other interspersed repeat elements in the genome. Gene model prediction and functional annotation Gene models were predicted for the repeat-masked genome using an evidence-based approach in MAKER [56] , which combines ab initio modelling with RNA-seq and protein sequence evidence ( Supplementary Note 8 ). Ab initio gene prediction was performed with SNAP [57] . Protein data consisted of all Arthropoda proteins from UniProtKB (UniProt release 2012_02) and whole proteomes of four species from Ensembl and two unpublished proteomes. As RNA-seq data, we used de novo -assembled transcripts [58] and TopHat/Cufflinks [59] mappings ( Supplementary Note 4 ). Noncoding and mtDNA genes were predicted as described in Supplementary Note 8 . Functional descriptions, gene ontologies and enzyme commission numbers were predicted for the protein sequences translated from the gene models and from the assembled transcripts using an in-house PANNZER annotation pipeline [60] ( Supplementary Fig. 14 ; Supplementary Note 8 ). Protein domains and other functional elements were detected and annotated using InterProScan [61] . Metabolic pathways and KEGG orthologues were predicted using the KAAS server [62] . Gene orthologies were predicted for the 5 lepidopteran species for which genome sequence information is available, 15 other arthropoda and 2 outgroups using an in-house EPT method [63] ( Supplementary Fig. 17 ). Variation analyses SNPs and indels were detected from four data sets as described in Supplementary Note 9 . The variation statistics described in the main paper are based on Illumina PE reads from a genomic pool of 10 full-sibs, which were also used in the genome assembly. The reads were mapped to the genome using BWA [51] , and variants were detected using a GATK pipeline [64] . Long indels were detected using a PacBio genomic pool from 100 individuals ( Supplementary Table 1 ). PacBio reads were mapped onto genomic scaffolds with BWA-SW [51] and indels exceeding 50 bp were detected. Linkage disequilibrium ( r 2 ) was estimated from the Illumina RNA-seq data for the population in the Åland Islands (Finland) using an in-house script ( Supplementary Fig. 25 ; Supplementary Note 9 ). Phylogenetic analyses The phylogenetic analyses were based on 312 species of the family Nymphalidae for which chromosome number and DNA sequences of 3–11 genes were available ( Supplementary Note 11 ). DNA sequences were manually aligned, and a phylogenetic hypothesis was inferred in the maximum likelihood framework using RAxML [65] . The haploid chromosome numbers were mapped onto the tree using Mesquite ( http://mesquiteproject.org ). Genome scans and synteny analyses GC, gene and repeat contents were calculated within 100 kb sliding windows and 10 kb shifts for the superscaffolds of M. cinxia and the genome sequence of B. mori [16] ( Supplementary Note 10 ). Since the superscaffolds were not ordered within bins in the current linkage map, the order and orientation of the superscaffolds within each bin were determined based on synteny to B. mori . Chromosome mapping was carried out using orthologous genes between M. cinxia and B. mori and between M. cinxia and H. melpomene to define the level of gene conservation and translocations among chromosomes ( Supplementary Notes 11 and 12 ). Furthermore, the mapped genes were used for the identification of fusion chromosomes in B. mori and H. melpomene . The same data set was used for calculating the number of breakpoints in the chromosomes, which were scaled by the number of one-to-one orthologues in the chromosomes, and used to measure the intrachromosomal rearrangement rate. Pairwise correlations between rearrangement rate, repeat content and chromosome lengths were calculated using the Pearson correlation coefficient. Chromosome mappings ( Fig. 2 ) are illustrated using Circos [66] . Possible bias in the ancestral chromosomes that are involved in fusion events in B. mori and H. melpomene was measured as follows. First, the probability for the same six ancestral chromosomes to be involved in independent fusions in both species was calculated as We assumed that B. mori has 6 and H. melpomene 20 fusion chromosomes, and each ancestral chromosome fused only once. Second, we measured the bias towards small ancestral chromosomes being involved in these fusions. The ancestral ( M. cinxia ) chromosomes were ranked according to chromosome number, which reflects the length ( M. cinxia chromosomes are numbered from the largest to the smallest). The median rank is 28 for B. mori and 18.5 for H. melpomene . The probabilities of obtaining at least as large medians by chance are 0.00092 and 0.14, respectively. The former is the probability of obtaining either chromosomes 28–31, or 27 and 29–31 from randomly chosen 6 chromosomes (out of 31), thus The latter probability was computed by simulating random draws of 20 chromosomes (out of 31). These P values were combined by Fisher’s method [67] to obtain the single P value of 0.0013. The approximate fusion sites were detected by aligning the fusion chromosomes of B. mori (11, 23 and 24) against the orthologous chromosomes of M. cinxia (12+31, 14+30 and 27+29) using Mauve [68] ( Supplementary Note 12 ). The content of TEs within the potential fusion regions was compared with the genome-wide content using RepeatMasker-open-4-0-2 with B. mori- and H. melpomene -specific repeat libraries [10] , [16] . Chromosome fusions in Fig. 5 and Supplementary Fig. 36 are visualized using in-house scripts. The annotated genome will be included in the EnsemblMetazoa http://metazoa.ensembl.org/Melitaea_cinxia/Info/Index . Further information, including superscaffolds, linkage map and annotations are available through our website at http://www.helsinki.fi/science/metapop/research/mcgenome.html . Accession codes : The genome sequence of the Glanville fritillary butterfly, Melitaea cinxia, has been deposited in DDBJ/EMBL/GenBank nucleotide core database under the accession code APLT00000000 . How to cite this article: Ahola, V. et al. The Glanville fritillary genome retains an ancient karyotype and reveals selective chromosomal fusions in Lepidoptera. Nat. Commun. 5:4737 doi: 10.1038/ncomms5737 (2014).